Nanoparticle exposure in animals can be visualized in the skin and analysed via skin biopsy The increasing use of nanomaterials raises concerns about the long-term effects of chronic nanoparticle exposure on human health. However, nanoparticle exposure is difficult to evaluate non-invasively using current measurement techniques. Here we show that the skin is an important site of nanoparticle accumulation following systemic administration. Mice injected with high doses of gold nanoparticles have visibly blue skin while quantum dot-treated animals fluoresce under ultraviolet excitation. More importantly, elemental analysis of excised skin correlates with the injected dose and nanoparticle accumulation in the liver and spleen. We propose that skin analysis may be a simple strategy to quantify systemic nanoparticle exposure and predict nanoparticle fate in vivo . Our results suggest that in the future, dermal accumulation may also be exploited to trigger the release of ultraviolet and visible light-sensitive therapeutics that are currently impractical in vivo due to limits in optical penetration of tissues at these wavelengths. Although the specific mechanisms are debated, most researchers agree that continuous intentional or unintentional exposure to nanomaterials can lead to chronic nanoparticle toxicity [1] . The measurement of nanoparticle exposure has been difficult because current quantification techniques require the isolation or sampling of internal organs [2] , [3] , [4] . These invasive and endpoint measurement methods are inappropriate for assessing nanoparticle accumulation in humans. Techniques using fluorescent and radio imaging modalities, such as whole-animal imaging [5] , [6] , raman spectroscopy [7] , multi-photon spectroscopy [8] and confocal microscopy [9] , have been employed in academic research for noninvasive measurement of nanoparticles in the skin. 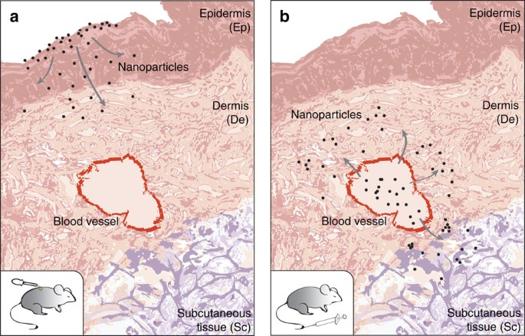Figure 1: Illustration of the routes of nanoparticle entry into the skin. (a) Nanoparticles applied topically to the outer surface of the mouse have been shown in previous studies to diffuse through the epidermis to reach the dermal (De) and subcutaneous (Sc) layers of the skin. (b) Systemic administration of nanoparticles by tail-vein injection was found in this study to enter the skin from blood vessels and diffuse into the De and Sc layers of the skin. Our study is focused on the systemic administration and not on the topical application as systemic administration is the most common method for introducing nanoparticle-based drugs and contrast agents into the body. Unfortunately, such methods only provide a semi-quantitative measure of the pharmacokinetic distribution of nanoparticles in organs and are limited to particles with specialized labels or properties that allow for detection ( Supplementary Table 1 ). Furthermore, detecting nanoparticles with such techniques has been difficult clinically due to the physical limitations of the required optical equipment. Quantitative and endpoint invasive techniques such as elemental analysis are capable of measuring nanoparticle biodistribution in small animals. Application of such modalities to humans has been limited [3] , [10] , [11] . To date, biodistribution analysis has been used to identify specific organs that are heavily exposed to nanoparticles. Such studies have shown that nanoparticles have a high propensity for accumulation in the liver and spleen. Despite being the largest vascularized organ of the body and an important component of the immune system, nonspecific skin accumulation of blood-circulating nanoparticles has only been mentioned in a handful of biodistribution studies [6] , [12] , [13] . Rather, skin nanomaterial research has been focused on assessing skin penetration and accumulation of topically applied nanoparticles composed of titanium oxide [8] , [14] , zinc oxide [15] and quantum dots [16] ( Fig. 1a ). In these studies, nanoparticles were applied to the skin and monitored by dermal microscopy [6] . This body of work has clearly shown that nanoparticles can permeate through hair follicles [17] , [18] and transiently extravasate from dermal blood vessels in vitro [19] . However, a thorough examination of the visual appearance and accumulation kinetics of blood-circulating nanoparticles in the skin after systemic injection ( Fig. 1b ) has yet to be conducted. Figure 1: Illustration of the routes of nanoparticle entry into the skin. ( a ) Nanoparticles applied topically to the outer surface of the mouse have been shown in previous studies to diffuse through the epidermis to reach the dermal (De) and subcutaneous (Sc) layers of the skin. ( b ) Systemic administration of nanoparticles by tail-vein injection was found in this study to enter the skin from blood vessels and diffuse into the De and Sc layers of the skin. Our study is focused on the systemic administration and not on the topical application as systemic administration is the most common method for introducing nanoparticle-based drugs and contrast agents into the body. Full size image Here, we show that intravenously administered inorganic nanoparticles at high doses are visible on the skin of mice under ambient light or through the use of inexpensive handheld devices such as ultraviolet lamps or dermatoscopes. We further show that elemental analysis of small skin biopsies can be used as a generalized approach to quantify the accumulation of gold nanoparticles and quantum dots within the body without the need of fluorescent or radioactive labels. Detection of gold nanoparticles in mouse skin Gold nanoparticles are commonly used in molecular diagnostics and drug delivery applications. These nanomaterials were selected for our initial studies as they are easily synthesized, have a distinct ruby colour and can be quantified by inductively coupled plasma atomic emission spectroscopy (ICP-AES). CD-1 nude athymic mice were tail-vein injected 15-nm gold nanoparticles functionalized with the anti-fouling polymer—methoxy-terminated polyethylene glycol (mPEG) and monitored for 21 days post injection (DPI). Coatings of mPEG were selected to lengthen plasma retention of injected nanoparticles by minimizing the adsorption of serum proteins and for its ubiquitous use in nanomedicine. Table 1 and Supplementary Fig. 1 summarize the characteristics of the functionalized nanoparticles used in our study. We observed that the complexion of mice injected with a minimum of 6.64 pmol of gold nanoparticles per gram body weight (gBW) turned from pink to blue after 24 h and persisted for 21 days ( Fig. 2a , Supplementary Fig. 2 , and Supplementary Movie 1 ). A similar change in skin colour was seen for nanoparticles coated with transferrin ( Fig. 2b ) as well as for 100 nm nanoparticles ( Fig. 2c ), indicating that the accumulation was not a size- or mPEG-specific phenomenon. Repeated dosing with 0.07 pmol gBW −1 of nanoparticles every other day also led to a change in skin colour 5 DPI ( Supplementary Fig. 3 ). This further implies that the nanoparticle-related changes in complexion were associated with retention of nanoparticles within the skin and not a byproduct of an excessively large bolus injection. Table 1 A summary of the physical properties of methoxy-terminated polyethylene glycol (mPEG)-functionalized nanoparticles. 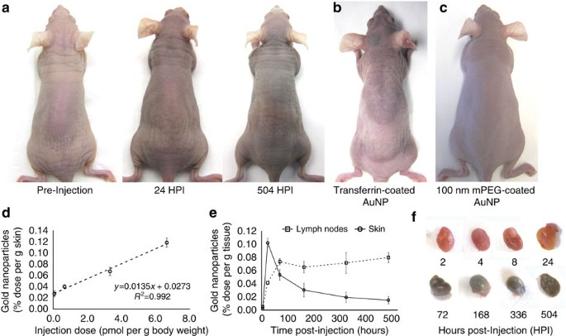Figure 2: Mice injected with gold nanoparticles. (a) Mice have a visible blue-purple complexion after tail-vein injection with 6.64 pmol of 15-nm gold nanoparticles functionalized with mPEG after 24 and 504 h post injection (HPI). (b,c) show the same skin discoloration when injected with 6.64 pmol of 15-nm gold nanoparticles functionalized with transferrin and 100-nm gold nanoparticles functionalized with mPEG, respectively. Inductively coupled plasma atomic emission spectroscopy ICP-AES was also used to measure the concentration of the gold nanoparticles. (d) A comparison of gold nanoparticle concentration in small skin biopsies (1.5 cm2) versus injection dose shows a direct correlation, while kinetic plots tracking gold nanoparticle concentration in the skin and lymph nodes (e) demonstrates that nanoparticle clearance from the skin (solid) coincides with an increase in nanoparticle concentration in the axillary lymph nodes (dotted). This suggests that the nanoparticles are cleared from the skin through the lymphatic system. Nanoparticle clearance from the skin levels off at 1.7% dose per gram tissue. (f) Isolated axillary lymph nodes show the gradual accumulation of gold nanoparticles (purple) in the lymph node over time. All error bars denote s.e.m. values for measurements (n>3). HPI, hours post-injection; AuNP, gold nanoparticle. Full size table Figure 2: Mice injected with gold nanoparticles. ( a ) Mice have a visible blue-purple complexion after tail-vein injection with 6.64 pmol of 15-nm gold nanoparticles functionalized with mPEG after 24 and 504 h post injection (HPI). ( b , c ) show the same skin discoloration when injected with 6.64 pmol of 15-nm gold nanoparticles functionalized with transferrin and 100-nm gold nanoparticles functionalized with mPEG, respectively. Inductively coupled plasma atomic emission spectroscopy ICP-AES was also used to measure the concentration of the gold nanoparticles. ( d ) A comparison of gold nanoparticle concentration in small skin biopsies (1.5 cm 2 ) versus injection dose shows a direct correlation, while kinetic plots tracking gold nanoparticle concentration in the skin and lymph nodes ( e ) demonstrates that nanoparticle clearance from the skin (solid) coincides with an increase in nanoparticle concentration in the axillary lymph nodes (dotted). This suggests that the nanoparticles are cleared from the skin through the lymphatic system. Nanoparticle clearance from the skin levels off at 1.7% dose per gram tissue. ( f ) Isolated axillary lymph nodes show the gradual accumulation of gold nanoparticles (purple) in the lymph node over time. All error bars denote s.e.m. values for measurements ( n >3). HPI, hours post-injection; AuNP, gold nanoparticle. Full size image Complementing our qualitative observation of nanoparticle accumulation, ICP-AES measurements seen in Fig. 2d of excised skin 24 h post injection (HPI) indicated that nanoparticle accumulation was linearly related to injection dose for concentrations between 0.07–6.64 pmol gBW −1 . Measurements of nanoparticle content in blood ( Supplementary Fig. 4 ) also confirmed that the nanoparticles measured in skin samples were representative of skin accumulation and not nanoparticles circulating in superficial blood vessels. The kinetics for our highest injection dose revealed that skin retention of our blood-circulating nanoparticles peaked at 24 HPI and decreased to a plateau concentration of 1.7±0.6% dose per g skin over 21 days ( Fig. 2e ). This decrease coincided with a cumulative increase of nanoparticles in the axillary, brachial and inguinal lymph nodes at 72 HPI ( Fig. 2f ). As dendritic cells are replaced from the dermis every 72 h (ref. 20 ), our findings imply that skin-accumulating nanoparticles are partially cleared by transport to the lymphatic system and affirm that the observed skin colour change was directly associated with nanoparticles rather than the permanent hyperpigmentation caused by elemental ions [21] , [22] , which are known to chelate with melanin [23] and accumulate dermally in patients afflicted with argyria [24] and chrysiasis [25] . The fate of gold nanoparticles within the lymphatic system remains unclear and will be investigated in future studies. Identification of skin layers that retain nanoparticles To further understand how gold nanoparticles became visible in the skin, histopathology was employed to visualize the location of nanoparticle accumulation. As illustrated in Fig. 3 , the skin is a stratified tissue that consists of an outer epidermal layer, a vascularized dermal layer and an insulating subcutaneous layer. Skin samples were harvested from mice at different time points between 4 and 504 HPI, histologically sectioned, and silver stained for visualization of nanoparticles. Using immunohistochemical stains for the F4/80 membrane marker for phagocytic cells [26] ( Fig. 3a ), we confirmed that nanoparticles accumulated in dermal macrophages and dendritic cells at low administration doses (0.07 pmol gBW −1 ). At higher treatments (0.67–6.67 pmol gBW −1 ), nanoparticles were seen in the pericellular space of the dermis and subcutaneous tissue ( Fig. 3b ). 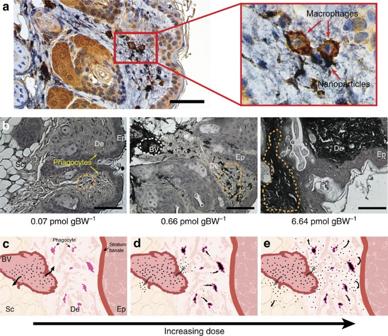Figure 3: Histology of skin samples post injection of gold nanoparticles at 20 × magnification. (a) Immunohistochemistry-stained skin section shows that macrophages (seen in brown) colocalize with nanoparticles (seen in black). Magnified inset clearly shows that nanoparticles can be found in the cytosolic region of macrophages. (b) Microscopy images demonstrate that as injected dose increases, nanoparticles (seen in black) appear to first localize in phagocytic cells (yellow arrow) then gradually begin to spill into the pericellular space of the dermis and finally distribute throughout the dermis (De) and subcutaneous tissue (Sc). Orange dotted lines highlight areas of nanoparticle accumulation. Nanoparticles were not detected in the epidermis (Ep) of the skin. Illustration panel (c–e) shows a pictorial diagram of nanoparticle infiltration into the skin over time. Post injection, nanoparticles begin to diffuse out of dermal blood vessels (BV) (c) and become taken up by dermal macrophages and dendritic cells (phagocytes) (d). Once phagocytic cells become saturated (e), nanoparticles begin to distribute into the pericellular space of the Subcutaneous tissue (Sc) and Dermis (De). Scale bars denote 50 and 200 μm for panels (a) and (b), respectively. gBW, gram of body weight. Figure 3c–e provide consecutive illustrations of the dose-dependent accumulation of nanoparticles within the skin. The visualization of nanoparticles in phagocytic cells and the pericellular space helps to explain the blue skin colour seen in mice as the high-packing density of gold nanoparticles in such regions and macrophage vesicles [27] can cause gold nanoparticle absorbance to visibly shift from red to blue [28] . Our histology also suggests that nanoparticle accumulation in the pericellular space occurs after cellular uptake of nanoparticles becomes saturated. Using both bright field microscopy ( Fig. 3b ) and transmission electron microscopy ( Supplementary Fig. 5 ) of skin sections, we determined and confirmed that the nanoparticles accumulating in the skin were not degraded in the dermis and did not penetrate into the epidermis of this skin. Nanoparticles are known to cross from the epidermis to the dermis when topically applied to the skin. Our results suggest that nanoparticle transport across the basal membrane is unidirectional whereby systemically administered nanoparticles do not cross the stratum basale for shedding during epidermal turnover [29] , [30] in the absence of physical damage to the skin or inflammation after skin accumulation [31] , [32] . Figure 3: Histology of skin samples post injection of gold nanoparticles at 20 × magnification. ( a ) Immunohistochemistry-stained skin section shows that macrophages (seen in brown) colocalize with nanoparticles (seen in black). Magnified inset clearly shows that nanoparticles can be found in the cytosolic region of macrophages. ( b ) Microscopy images demonstrate that as injected dose increases, nanoparticles (seen in black) appear to first localize in phagocytic cells (yellow arrow) then gradually begin to spill into the pericellular space of the dermis and finally distribute throughout the dermis (De) and subcutaneous tissue (Sc). Orange dotted lines highlight areas of nanoparticle accumulation. Nanoparticles were not detected in the epidermis (Ep) of the skin. Illustration panel ( c – e ) shows a pictorial diagram of nanoparticle infiltration into the skin over time. Post injection, nanoparticles begin to diffuse out of dermal blood vessels (BV) ( c ) and become taken up by dermal macrophages and dendritic cells (phagocytes) ( d ). Once phagocytic cells become saturated ( e ), nanoparticles begin to distribute into the pericellular space of the Subcutaneous tissue (Sc) and Dermis (De). Scale bars denote 50 and 200 μm for panels ( a ) and ( b ), respectively. gBW, gram of body weight. Full size image Effect of gold nanoparticles on animal toxicity We next sought to determine whether the doses required for visible detection of gold nanoparticles in mouse skin were associated with animal toxicity. The health of mice injected with gold nanoparticles at a dose of 6.67 pmol gBW −1 was monitored at 7 and 21 DPI to assess the upper threshold of nanoparticle toxicity for our study. Mouse health was closely monitored for signs of distress and changes to body weight. By appearance, mice administered with gold nanoparticles were normal and did not significantly drop in body weight compared with control animals injected with phosphate-buffered saline ( Supplementary Fig. 6 ). Blood biochemistry and haematological analysis were also performed to assess systemic toxicity in our mice. A brief description of the parameters used for blood biochemistry and haematological analysis is summarized in Supplementary Tables 2 and 3 , respectively. White blood cell count, monocyte, neutrophil and lymphocytes ( Supplementary Fig. 7 ), were universally below the health range specified by the breeder, Charles River laboratories ( www.criver.com/files/pdfs/rms/cd1-nude/rm_rm_r_cd-1_nude_mouse_clinical_pathology_data.aspx ). However, the similarity between nanoparticle-treated and untreated mice suggests that the sub-standard readings were likely related to mouse age and stress versus nanoparticle exposure [33] . Acute liver toxicity was estimated by quantification of haematological enzyme levels ( Supplementary Fig. 8 ). Once again, our values were below those reported by the breeder specifications but not statistically different from control groups. Acute liver toxicity is typically associated with significant elevation in bilirubin [34] , alkaline phosphatase [33] , alanine aminotransferase [35] and aspartate aminotransferase [35] . These enzyme levels can fluctuate due to an animal’s level of physical activity as well as the time of day in which blood was sampled [33] . Hence, we concluded that the universally lower values for both treatment and control groups were likely not associated with nanoparticle toxicity. We, however, would like to note that although gold nanoparticle toxicity was not observed at the reported doses, our toxicology results may not predict the long-term impact of nanoparticle exposure on healthy animals and may not be generalizable to other nanoparticle types as particle composition and surface chemistry may yield different biological effects. Influence of quantum dots on mouse skin Building on our gold nanoparticle observations, we explored whether skin accumulation occurred for other nanoparticle types. To test, we injected mice with mPEG-functionalized quantum dots at doses similar to gold nanoparticles by normalizing to total nanoparticle surface area (4.4–80 pmol gBW −1 ). Three alloyed quantum dots (ZnS-capped, CdSeS) with distinct fluorescent emissions (525, 575 and 667 nm) were chosen to demonstrate the range of visually detectable colours. The injection of quantum dots did not adversely impact mice ( Supplementary Movies 1 and 2 ) at all administered doses. Unlike gold nanoparticles, the skin colour of quantum dot administered animals did not change under white light illumination. This is likely related to the quantum dot’s lower extinction coefficient in comparison with gold nanoparticles [36] , [37] . We alternatively observed that the animals fluoresced green, yellow and red under ultraviolet lamp illumination corresponding to the spectral properties of the injected quantum dots ( Fig. 4a ). These ultraviolet-dependent changes further validated that the nanoparticles, and not their free metal ions accumulated in the skin as quantum dots lose their fluorescence with particle degradation [38] . We observed that the quantum dots that fluoresced green and yellow were more pronounced in the mouse skin than red-emitting formulations. This was likely related to the higher quantum yield of green and yellow quantum dots that allowed them to be visible over the absorption and scattering properties of the dermis [39] , [40] . 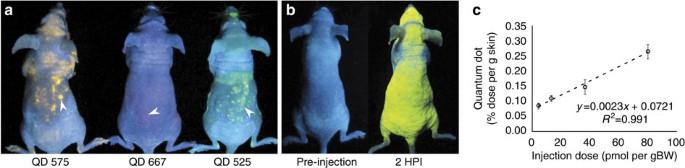Figure 4: Mice injected with quantum dots. (a) Mice injected with quantum dots of different emission wavelengths (575, 667 and 525 nm) were simultaneously imaged at 2 HPI under a handheld ultraviolet light illumination. White arrows delineate points of quantum dot accumulation. (b) An example of a mouse pre- (left) and post (right) injection of quantum dots where fluorescence covers the entire skin. (c) ICP-AES quantification of quantum dots in the skin was also linearly related to injection dose at 72 HPI. Error bars denote s.e.m. for measurements (n>3). QD refers to quantum dots and the number corresponds to the wavelength of maximum fluorescence emission. bBW refers to gram of body weight. Figure 4: Mice injected with quantum dots. ( a ) Mice injected with quantum dots of different emission wavelengths (575, 667 and 525 nm) were simultaneously imaged at 2 HPI under a handheld ultraviolet light illumination. White arrows delineate points of quantum dot accumulation. ( b ) An example of a mouse pre- (left) and post (right) injection of quantum dots where fluorescence covers the entire skin. ( c ) ICP-AES quantification of quantum dots in the skin was also linearly related to injection dose at 72 HPI. Error bars denote s.e.m. for measurements ( n >3). QD refers to quantum dots and the number corresponds to the wavelength of maximum fluorescence emission. bBW refers to gram of body weight. Full size image Interestingly, the distribution of fluorescence in the mouse skin was dose-dependent. Mice uniformly fluoresced at an injection concentration of 240 pmol gBW −1 ( Fig. 4b ) but were patchy at lower quantum dot doses. In some animals, fluorescence was observed in one ear and not the other or in varied regions of the body ( Supplementary Movies 1 and 2 ). The cause for the non-uniform distribution of fluorescence is unclear, but may be related to the location of phagocytic cells, differences in the superficial vasculature or depth of accumulation. Nevertheless, skin fluorescence was detectable as early as 2 HPI in all cases but gradually faded over 24–36 h ( Supplementary Fig. 9 ). Ultraviolet B light (290–320 nm) fails to penetrate beyond the epidermis and ultraviolet A light (320–400 nm) is limited to dermal permeation. Particles residing deeper in the dermis and subcutaneous tissue would be more difficult to detect visually [39] . We suspect that the fluorescent fading is related to particle movement from more superficial regions to deeper layers. This was further validated by ICP-AES measurement ( Fig. 4c ) and histological analysis ( Supplementary Fig. 9 ) of skin biopsies, which demonstrated that quantum dots remained present in the skin at a higher concentration than in blood 72 HPI ( Supplementary Fig. 4 ). Despite their complete loss of visual fluorescence, presence of quantum dots in the skin remained linearly correlated to the injection dose similar to the results for gold nanoparticles ( Fig. 4c ). This reinforces the idea that nanoparticle accumulation in the skin is independent of particle-type and intimates that nanoparticles with an optical or magnetic emission (most inorganic nanoparticles) may be detected by visual changes in skin tone. Correlation of skin accumulation to the liver and spleen Since skin retention of nanoparticles was seen to be dose-dependent, we investigated whether such dermal measurements could be used to predict nanoparticle accumulation in other organs of the body. High quantities of nanoparticles are known to sequester in the liver and spleen [27] , [41] . This high retention can make these organs particularly susceptible to toxicity caused by nanoparticles. Unfortunately, the only strategy to assess nanoparticle exposure in these tissues is organ sampling. This technique can be undesirable, as it can expose the body to infection and may lead to decreased organ function. We opted to test whether minimally invasive skin punctures—a common clinical technique [42] —taken from the central region on the dorsal side of mice could be used to measure internal organ exposure to nanoparticles. The limit of detection of nanoparticles in the skin by ICP-AES was evaluated by spiking standard dilutions of gold nanoparticles and quantum dots with mouse skin. We identified that gold nanoparticles and quantum dots could be detected down to 0.04 and 0.028 pmol, respectively ( Supplementary Fig. 10 ). Interestingly, liver and spleen accumulation of gold nanoparticles ( Fig. 5a,b ) at 24 HPI and quantum dots ( Fig. 5c,d ) at 72 HPI were linearly related to the injected dose. We further noticed that nanoparticle content in these organs could be predicted by multiplying the measured nanoparticle content in the skin by a constant for all administered doses ( Fig. 5e,f ). This relationship between the skin, liver and spleen implies that skin biopsies can be used as an easily accessible and minimally invasive surrogate measure of reticuloendothelial organ exposure to nanoparticles. This may conceivably be useful for clinical identification of the type and degree of nanoparticle exposure in the future. 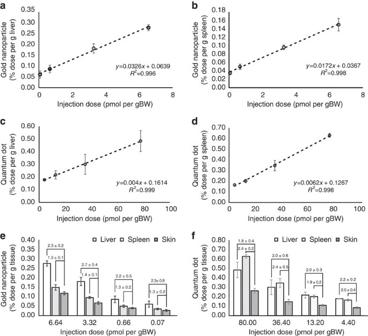Figure 5: ICP-AES analysis of organs post nanoparticle administration. (a,b) Accumulation of 15 nm gold nanoparticles in the liver and spleen at 24 HPI was linearly related to injection dose. (c,d) Accumulation of quantum dots in the liver and spleen at 72 HPI was also linearly related to injection dose. (e,f) As the injection dose decreases, we observed a corresponding decrease in the amount of nanoparticles in the liver, spleen and skin. Interestingly, the quantity of the gold nanoparticles and quantum dots in the liver and spleen was directly related to the skin. This suggests that we can estimate the amount of nanoparticles in the other reticuloendothelial organs by multiplying skin measurements by a numeric factor. For example, the concentration of gold nanoparticles in the liver for an injection dose of 6.64 pmol per g body weight can be obtained by multiplying the measured skin quantity by 2.3. We confirmed that the ratios are statistically similar, using the student’st-test (P>0.05). Injection doses for gold nanoparticle and quantum dots were normalized to total surface area to compare between particle types. Error bars denote s.e.m. for measurements (n>3). Figure 5: ICP-AES analysis of organs post nanoparticle administration. ( a , b ) Accumulation of 15 nm gold nanoparticles in the liver and spleen at 24 HPI was linearly related to injection dose. ( c , d ) Accumulation of quantum dots in the liver and spleen at 72 HPI was also linearly related to injection dose. ( e , f ) As the injection dose decreases, we observed a corresponding decrease in the amount of nanoparticles in the liver, spleen and skin. Interestingly, the quantity of the gold nanoparticles and quantum dots in the liver and spleen was directly related to the skin. This suggests that we can estimate the amount of nanoparticles in the other reticuloendothelial organs by multiplying skin measurements by a numeric factor. For example, the concentration of gold nanoparticles in the liver for an injection dose of 6.64 pmol per g body weight can be obtained by multiplying the measured skin quantity by 2.3. We confirmed that the ratios are statistically similar, using the student’s t -test ( P >0.05). Injection doses for gold nanoparticle and quantum dots were normalized to total surface area to compare between particle types. Error bars denote s.e.m. for measurements ( n >3). Full size image Effect of tissue origin on nanoparticle quantification As a final task, we validated whether nanoparticle quantification of the skin by ICP-AES was consistent across different regions of the body and independent of species. Nanoparticle content in skin samples taken dorsally from gold nanoparticle-treated mice at the cranial, central and caudal regions and was compared by ICP-AES. Despite the visual inhomogeneity of skin accumulation, nanoparticle content was statistically uniform ( Supplementary Fig. 11 ). This both indicated that (i) the patchy pigmentation was likely caused by nanoparticle accumulation at deeper layers of the skin and (ii) skin biopsies can be taken from anywhere on the body for ICP-AES measurement. Measurement of nanoparticle content in the skin versus blood ( Supplementary Fig. 4 ) further confirmed that the concentration of nanoparticles in the skin was reflective of tissue accumulation and not nanoparticle presence within superficial blood vessels of the skin. We also examined whether the measurements of excised skin were biased by the animal species to ensure that ICP-AES measurement of skin samples could be translated for use with nonmouse tissues. Standard dilutions of gold nanoparticles and quantum dots were spiked with samples of porcine, rabbit and mouse skin. Our results demonstrated that nanoparticle measurement was unaffected by the presence of skin from different animals ( Supplementary Fig. 10 ) and validated that ICP-AES analysis of skin biopsies could potentially be used for the assessment of nanoparticle exposure in human tissues. In light of the growing interest in nanomedicine, the observation of nanoparticle accumulation in the skin is significant from a number of perspectives. First, it demonstrates that systemic exposure to inorganic nanoparticles can be detected by visual and elemental analysis of the skin. The ability to use skin to determine exposure provides a noninvasive and rapid determination of nanoparticle exposure that can be further quantified by ICP-AES after skin biopsy. This quantification method addresses the need for an absolute nanoparticle quantification scheme that is unencumbered by the interference from biological tissues which commonly limit noninvasive optical detection techniques such as two-photon or Raman microscopy (see Supplementary Table 1 for comparison). Second, our observations allude to the need for further study of the toxicological impact of nanomaterials on the skin. Skin accumulation of nanoparticles postsystemic administration may result in the adverse generation of reactive oxygen species or heat through low tissue-penetrating ultraviolet or visible light excitation. This will become increasingly important as nanomaterials become incorporated into commercial products and industrial processes. On the bright side, our findings suggest that nanoparticle accumulation in the skin may also be exploited to develop novel strategies for engineering photoresponsive nanomaterials for diagnosing diseases or for controlling drug release via systemic injection (unpublished data). Although our work demonstrates that nanoparticles accumulate in the skin, the observed differences in the kinetics of skin accumulation between the gold nanoparticles and quantum dots suggest that additional investigation into different nanoparticle sizes, shapes, surface chemistries and routes of administration is required to identify how the physico-chemical properties of a nanoparticle and modes of exposure may affect their skin accumulation. Such work will provide a better understanding of the biodistribution behaviour of nanoparticles in vivo and will allow for the exploitation of dermal accumulation for practical use. Despite the need for future studies, our current findings shed new light on the accumulation patterns of nanomaterials in vivo and also provide a wealth of new opportunities for engineering novel diagnostics and therapeutics using optical wavelengths with low tissue penetration. Nanoparticle synthesis and functionalization Fifteen-nanometre gold nanoparticles were synthesized by methods described previously by Frens et al . [43] In short, 100 ml of double-distilled water was set to boil with 0.3 mg ml −1 of sodium citrate tribasic (Sigma S4641), followed by the addition of 9.85 mg of gold (III) chloride trihydrate (Sigma G4022) under rapid stirring and reflux for 7 min. Citrate-stabilized gold nanoparticles were concentrated and surface functionalized with 5 kDa sulfhydryl-mPEG (Laysan Bio MPEG-SH-5000) at an excess reaction ratio of four methoxy-terminated polyethylene glycol nm −2 under heated conditions (60 °C) for 30 min. Trilite Quantum dots with fluorescent emissions of 525, 575 and 667 nm were purchased from CytoDiagnostics, Burlington, Canada and functionalized with 5 kDa sulphydryl-mPEG groups using a two-step ligand exchange. Briefly, chloroform-solubilized quantum dots were mixed with thioglycolic acid (Sigma T3758) under stirring conditions for 5 h at room temperature and washed in acetone containing 1.85% wt v −1 tetramethylammonium hydroxide pentahydrate (Sigma T7505). Quantum dots were then reacted with sulphydryl-mPEG in 50 mM borate buffer at a 1:11250 ratio at 60 °C for 60 min followed by Amicon ultracentrifuge tube (Millipore UFC5030) purification. Hydrodynamic diameter and zeta potential of nanoparticles were determined by dynamic light scattering using a Malvern Nano ZS in 10 mM HEPES buffer spiked with 3 mM sodium hydroxide and 1 ml sodium chloride. Nanoparticle core-diameters were measured by transmission microscopy, while functionalization was validated by gel-shift in 0.7% wt v −1 agarose gels at 135 mV for 15 min. Dose preparation and animal injection Four-week-old female CD-1 nude athymic mice were purchased from Charles River and maintained in the Division of Comparative Medicine, University of Toronto. For dose preparation, mPEG-functionalized gold nanoparticles (0.2, 0.02 and 0.002 nmol) and quantum dots (0.11, 0.31, 0.91 and 2 nmol) were buffered to physiological pH in 1 × phosphate-buffered saline with a final volume of 200 μl. Doses were warmed to room temperature before gradual intravenous injection into 5–6-week-old mice over 1 min to minimize shock to the animals. Mice were monitored over the period of study for health complications and changes to body weight. All procedures were conducted in compliance with the ethical regulations set out by the Faculty of Medicine and Pharmacy Animal Care Committee, University of Toronto. Organ and blood collection Mice were warmed under heat lamp illumination for 30 min before blood collection. For blood half-life analysis, 10 μl of blood was collected by tail-vein puncture into EDTA-coated capillary tubes (Drummond Microcap 1-000-2000-E) at 2, 4, 8, 24, 48 and 72 HPI. Haematological samples were collected from mice via cardiac puncture at an extraction rate of 0.3 ml s −1, while anaesthetized with isofluorane-enriched oxygen. Blood biochemistry and haematology were processed by the Samuel Lunenfeld Research Institute to assess nanoparticle-related toxicity. Mice were then killed by cervical dislocation for organ and lymph node collection. Animal handling was performed in accordance with methods approved by the Faculty of Medicine and Pharmacy Animal Care Committee, University of Toronto. Tissue histology preparation Tissue samples were harvested from mice and immediately fixed in 10% buffered formalin for 7 days. Tissues were then paraffin-embedded and stained by the Department of Pathology at Toronto General Hospital. Haematoxylin and eosin were used for tissue contrast, while silver and F4/80 antibody (Serotec MCA497GA) were used to visualize nanoparticles and macrophages/dendritic cells, respectively. Briefly, tissues were stained with antibodies at a 1/20,000 dilution for 1 h, while silver stain was allowed to develop over 30 min. Following staining, slides were thoroughly washed in double-distilled water and imaged using an Olympus IX-70 inverted light microscope mounted with an Amscope MU500 camera at 10 × and 20 × magnification. Biodistribution analysis Tissues were digested in yttrium (1 μg ml −1 ) supplemented aqua regia (75% hydrochloric acid, 25% nitric acid) at 70 °C for 2 h. Digested organs were diluted in double-distilled water and filtered through Millipore 0.22 μm PVDF filters (Millex GV) to remove debris. Gold and cadmium content was quantified via ICP-AES (Perkin-Elmer Optima 3000) to determine organ concentration of gold nanoparticles and quantum dots, respectively. Yttrium was used as a reference to account for sample loss during tissue processing. All measurements were normalized to injection dose and wet tissue mass. Optical imaging of mice Whole-animal images were acquired while mice were anaesthetized with isofluorane-enriched oxygen using a Canon Powershot S95 camera. Gold nanoparticles were imaged under normal white light conditions, while quantum dot fluorescence was achieved through illumination with a handheld ultraviolet lamp. Images were acquired at 0.17, 2, 4, 8, 24, 48, 72, 168, 336 and 504 h post nanoparticle injection. How to cite this article : Sykes, E. A. et al . Nanoparticle exposure in animals can be visualized in the skin and analysed via skin biopsy. Nat. Commun . 5:3796 doi: 10.1038/ncomms4796 (2013).